Direct growth of aligned graphitic nanoribbons from a DNA template by chemical vapour deposition Graphene, laterally confined within narrow ribbons, exhibits a bandgap and is envisioned as a next-generation material for high-performance electronics. To take advantage of this phenomenon, there is a critical need to develop methodologies that result in graphene ribbons <10 nm in width. Here we report the use of metal salts infused within stretched DNA as catalysts to grow nanoscopic graphitic nanoribbons. The nanoribbons are termed graphitic as they have been determined to consist of regions of sp 2 and sp 3 character. The nanoscopic graphitic nanoribbons are micrometres in length, <10 nm in width, and take on the shape of the DNA template. The DNA strand is converted to a graphitic nanoribbon by utilizing chemical vapour deposition conditions. Depending on the growth conditions, metallic or semiconducting graphitic nanoribbons are formed. Improvements in the growth method have potential to lead to bottom-up synthesis of pristine single-layer graphene nanoribbons. Despite the recently reported outstanding electrical characteristics of graphene, the development of field-effect transistors (FETs) based on this semi-metal is not practical owing to a lack of a bandgap. The lateral confinement of the graphene structure within a narrow ribbon of widths <10 nm can result in the creation of a bandgap and provide a pathway towards high-performance FET devices. Several methods to confine graphene within nanoribbons of widths <10 nm have been reported. The methods include lateral unzipping of carbon nanotubes [1] , [2] , [3] , as well as plasma etching of graphene through masks prepared using nanospheres [4] , [5] , block copolymers [6] , [7] or lithographically [8] . In addition, three methods for the direct synthesis of nanoribbons have been reported including a bottom-up synthesis from molecular components [9] and an epitaxial growth from SiC utilizing the preferential precipitation of graphene from a pre-patterned facet [10] . However, these methods are limited in the dimensions of the resultant structures [11] . A scalable method for growth of aligned ribbons with widths <10 nm would have a significant impact on the development of next-generation high-performance electronic devices. Unfortunately, the direct growth of graphene nanoribbons presents several challenges. The main challenge is the localization of carbon atoms to the desired nanoscopic area of the target substrate during the growth. One recent method to achieve nanoribbon localization is the growth of graphene from the edge step of a thin metal film, achieving ribbon thicknesses <20 nm thus far [12] , [13] . A different strategy, used to localize carbon in two dimensions, is the conversion of a deposited carbonaceous material to graphene. There have been several literature reports that utilize solid carbon sources on metallic catalyst supports to result in single- and multi-layer graphene structures [14] , [15] , [16] . Graphitization of carbon layers has been previously demonstrated with the assistance of a thin film of a transition metal catalyst at high temperature [17] . In addition, metal ions have also been shown to catalyse the carbonization of bulk coordination polymers [18] , [19] . Recent reports have demonstrated that a crosslinked self-assembled monolayer can be converted into a graphitic structure utilizing a high-temperature anneal. The resulting 1 nm film demonstrated both graphitic and amorphous carbon domains [20] , [21] . However, in all cases, there is no demonstrated control of localization of graphene growth within one dimension to achieve nanoscale ribbons. This, one-dimensional localization is widely recognized as a significant challenge, owing to both carbon and metal catalyst migration [14] and evaporation at the required temperatures [22] , [23] . A recent paper has demonstrated that carbon atoms from a solid source, namely an insect leg, resulted in graphene formation on the underside of the copper film [14] . It was not clear if the carbon atom migrated through or around the copper film; however, the placement of the solid source was critical to graphene quality. When the carbon source was placed away from the metal foil, only an amorphous layer of carbon formed. This suggests that for graphene growth, the carbon migration on the catalyst foil was important. For these reasons, it is technologically difficult to achieve lateral confinement for graphitic structures in a controlled manner. The direct growth of graphene from a nanometre-wide metal catalyst template is not feasible, as the nanoscale lines would melt and de-wet during typical graphene chemical vapour deposition (CVD) conditions [22] , [23] . In this report, we describe the first steps towards the direct growth of nanoscale graphitic structures. We demonstrate that graphitic nanoribbons (GraNRs) can be directly synthesized from a solution-processed, aligned DNA template. To overcome the inherent limitation of nanoscale metals, we turned to metal salts as precursor catalysts. We hypothesized that an organic template impregnated with metal salts can form nanoscale features and prevent metal ion diffusion or de-wetting. The resulting GraNRs are <10 nm in width and exceed 20 μm in length. The materials are termed graphitic, owing to the mixed regions of crystalline graphene ( sp 2 ) and amorphous carbon ( sp 3 ) distributed throughout the ribbon. In this manner, we demonstrate the route towards the direct growth of ultrathin graphitic and potentially graphene nanoribbons. DNA templates and graphitization To achieve linear features with widths <10 nm, we chose DNA as our template. DNA can be easily stretched by molecular combing and has been used to form metal nanowires via the reduction of bound metal salts [24] . In this paper, we have focused on the use of Cu 2+ because copper has been demonstrated as a catalyst for single-layer graphene. In future work, additional metals will be investigated (for example, Ni and Co). 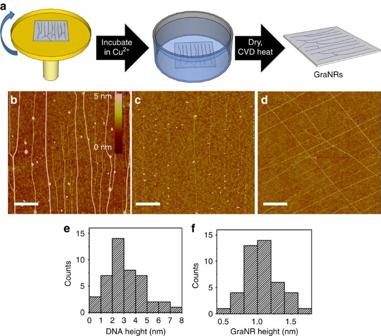Figure 1: Fabrication of GraNRs from DNA template. (a) Schematic process of DNA to GraNR conversion. AFM images of (b) DNAs stretched and aligned on the substrate, (c) GraNRs after SGP and (d) GraNR cross-bar architecture. Scale bar, 1 μm. Histograms of (e) DNA and (f) GraNR heights. The standard growth process (SGP) conditions and the mechanistic growth studies are outlined in Table 1 . Table 1 Summary of conditions performed for GraNR growth. Full size table To form the GraNRs from DNAs infused with metal ions, a solution of double-stranded lambda DNAs was spin-coated onto a substrate resulting in aligned DNAs stretching over 20 μm. Next, the DNAs were immersed into 0.1 M solution of Cu(NO 3 ) 2 infusing the DNAs with Cu 2+ ions ( Fig. 1a ). A concentration of 0.1 M Cu(NO 3 ) 2 was used to saturate the DNAs with Cu 2+ ions. Higher concentrations of Cu 2+ were avoided to prevent increased non-specific background adsorption. The influence of increased Cu 2+ concentrations on GraNR growth is the subject of ongoing investigations. The wafers were subsequently placed into a furnace and subjected to thermal treatments [25] . Figure 1: Fabrication of GraNRs from DNA template. ( a ) Schematic process of DNA to GraNR conversion. AFM images of ( b ) DNAs stretched and aligned on the substrate, ( c ) GraNRs after SGP and ( d ) GraNR cross-bar architecture. Scale bar, 1 μm. Histograms of ( e ) DNA and ( f ) GraNR heights. Full size image Figure 1b,c shows the typical atomic force microscopy (AFM) images of DNAs stretched on a substrate and the resulting GraNRs after SGP. Over hundreds of AFM images taken during growth optimization, the bundling, density and branching of the resultant GraNR structures clearly mimicked the DNA nanostructure shapes in the DNA template (see Supplementary Fig. S1 for more AFM images of GraNRs). Although for our applications, namely transistors, conditions providing long unbranched lines were chosen, the use of DNA-deposition conditions leading to increased curvature or branches resulted in GraNRs of similar structure. The height of over 40 DNAs are given in the histogram ( Fig. 1e ); they varied from <1 nm to 8 nm. As the height of a single dsDNA from AFM measurements was reported to be ~0.7 nm [26] , our stretched DNAs are likely bundles of several dsDNAs. It should be noted that because of DNA bundling and AFM tip sizes, the helical nature of the DNA could not be observed. The density, branching and bundling can be controlled by both DNA concentration and ionic strength [27] . The quantitative correlation of size to GraNR performance is a subject of follow-up work. After the SGP converts the DNAs into GraNRs, the heights of the structures were significantly reduced, ranging from ~0.5 to<2 nm ( Fig. 1f ). This suggests that the graphitization is accompanied by a significant atomistic re-arrangement, likely leading to a loss of helicity imparted by the DNA template. However, if helicity of the resulting ribbons could be observed, this would be of significant interest to the electronics community. AFM analysis suggests that the GraNRs are continuous over the 5-μm scan size ( Fig. 1c ). However, defects smaller than the curvature of the AFM tip would be difficult to detect by this method; thus, electrical conductivity measurements as means to establish continuity are discussed within the manuscript. The width of the GraNR measured between about 4.9 and 10 nm (see Supplementary Figs S2 and S3 ). To demonstrate the versatility of the approach, we fabricated GraNR cross-bar architectures ( Fig. 1d ). The structures were accessed by two stages of successive transfer printing of DNA lines onto a substrate, separately, by a~90 o rotation [28] , [29] . The cross-bar DNAs are infused with Cu 2+ ions and are converted to GraNRs with the CVD process. These cross-bar architectures demonstrate that the method is compatible with DNA stamping and printing techniques, allowing for successive patterning and directional control of the resultant GraNR architectures. Moreover, this clearly demonstrates that the GraNRs are templated by the direction and pattern of the DNA templates. The patterns may be used to increase current density, decrease performance variability in GraNR-based devices, as well as a possible first step towards the formation of graphene p–n junctions. As DNA is a highly versatile template for patterning, we anticipate that graphitic structures with unusual shapes can be rendered by using unique DNA templates, such as DNA origami [30] . XPS characterization of GraNR structures X-ray photoemission spectroscopy (XPS) was performed to study the elemental composition and carbon structure of DNA after thermal treatments. As the GraNR density using DNA bundles was too low to give sufficient XPS signal, we used DNA films that were subjected to exactly the same growth conditions while monitoring with XPS, AFM and Raman ( Fig. 2 and Supplementary Figs S4 and S5 ). The XPS spectra were analysed using a fitting routine to de-convolute each spectrum into individual mixed Gaussian–Lorentzian peaks, with their binding energy and percentage composition (see Supplementary Table S1 and Supplementary Fig. S6 ) [31] . To characterize the quality of the DNA-templated GraNRs, we utilized XPS to quantify the sp 2 to sp 3 ratio for each set of growth conditions. The sp 2 ratio was defined by the area under the curve of the peak fit at 284.5 eV, with the full-width half-maximum (FWHM) defined as 1.2 eV (refs 31 , 32 ). The sp 3 quantity was determined by the peak centred between 285.0 and 285.5 eV, with a variable FWHM. For the sp 3 peak, the FWHM was consistent, between 1.45 and 1.79 eV (refs 31 , 32 ). For each set of conditions, a peak at higher eV (287.6–288.1 eV), assigned to oxidized carbon atoms (C–O or C=O) was also fitted. However, for all conditions this peak accounted for approximately 15–20% of the total area and was not used in the overall comparison. As a standard, we characterized a CVD-grown single-layer graphene film transferred onto SiO 2 . The C1s peak of CVD graphene transferred onto SiO 2 exhibits approximately 85% sp 2 carbon content, typical for transferred CVD-grown graphene owing to defects and contamination arising during the transfer process [33] . We also characterize the as-cast DNA film, which did not exhibit a significant peak at 284.5 eV (<2.5% of overall area), but rather a broad C1s signal from the C–H, C–N, C–O and C=O bonds of the DNA [34] . The relative assignments of the sp 2 and sp 3 percentages are tabulated in Supplementary Table S1 . From the table, it is clear that the relative percentage of the sp 2 carbon is the highest for our SGP. Upon exposure to the SGP, the C1s peak of the DNA narrowed to a dominant sp 2 peak at 284.5 eV (58.2% sp 2 composition), indicating significant conversion to graphitic carbon. In contrast, DNA exposed to H 2 in the absence of CH 4 had only 38.4% sp 2 composition, whereas the DNA exposed to Ar exhibited only 12.9% sp 2 composition. In all cases, a significant amount of sp 3 carbon is present, with the amount increasing from 27.1 to 41.8% and finally to 71.2% for the SGP, H 2 and Ar conditions, respectively. The relative ratio of H 2 within the carrier gas has not been investigated; however, it has been shown in literature to make a significant impact on the growth mechanism of graphene [15] . 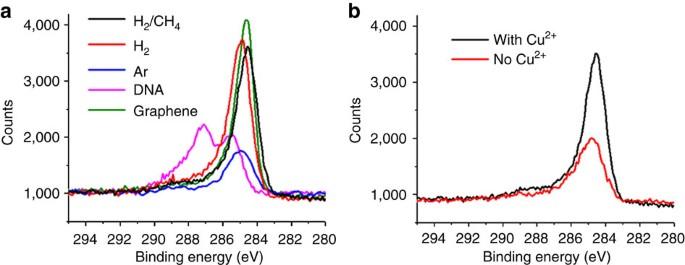Figure 2: High-resolution XPS spectra of the C1sregions for DNA. (a) DNA (magenta), transferred CVD graphene (green), DNA after Ar at 1,000 °C (blue), H2at 1,000 °C (red) and after the SGP (black). (b) DNA after SGP with (black) and without Cu2+(red). Figure 2: High-resolution XPS spectra of the C1 s regions for DNA. ( a ) DNA (magenta), transferred CVD graphene (green), DNA after Ar at 1,000 °C (blue), H 2 at 1,000 °C (red) and after the SGP (black). ( b ) DNA after SGP with (black) and without Cu 2+ (red). Full size image Next, we investigated the effect of infusing the DNA with Cu 2+ ( Fig. 2b , black). Exposing the DNA to SGP conditions without Cu 2+ ions resulted in a significant reduction of sp 2 composition from 58.2 to 32.8%. Moreover, the peak intensity was lower in the absence of Cu 2+ (ref. 15 ), suggesting that some DNA carbon atoms were removed. We hypothesize that the growth process involves reduction of Cu 2+ to Cu 0 by H 2 , which subsequently catalyses sp 2 carbon formation. The Cu 2+ to Cu 0 transition is evident from the shift in the Cu2p 3/2 peak from 934.2 to 932.5 eV when DNA infused with Cu 2+ was annealed to 600 °C in the presence of H 2 (see Supplementary Fig. S7a ). It should be mentioned that going through the SGP using the stretched DNAs on Cu foils did not result in the formation of observable GraNR structures, suggesting that in the absence of incorporated metal ions, the organic material either decomposes or migrates on the foil before graphitization [14] , [15] . The Cu 0 embedded within the carbon matrix acts as a catalyst to convert sp 3 carbons to sp 2 carbons in the presence of CH 4 . Following the SGP, Cu atoms were no longer detected. It is well documented in literature that significant evaporation of Cu occurs during graphene growth ( T Growth 800–1,000 o C) [23] . For our experiments, despite the minute amount of copper on our samples, copper deposition was observed at the ends of the fused silica tube following multiple growth experiments. Similarly, N or P could not be detected, suggesting the decomposition of the phosphodiester backbone (see Supplementary Fig. S7b,c ). Although this suggests that a majority of N and P is removed during the SGP, the method cannot quantitatively rule out the incorporation of N or P within the resulting GraNR structure. Previously, literature studies have demonstrated that a significant loss of nitrogen can occur from N-doped solids during a high-temperature annealing processes [16] . The incorporation of hetero-atoms resulting in deliberate doping of graphitic structures during growth is an exciting area for future nanoscale research. Raman characterization of GraNR structures Raman spectroscopy is a powerful tool to characterize graphene structures [35] , [36] . Our stretched DNAs did not exhibit a Raman signal ( Fig. 3a , magenta). Following SGP, two distinct peaks at 1,333 and 1,600 cm −1 were observed ( Fig. 3a , red). These are referred to as the D and G peak, respectively; they are two prominent features of sp 2 bonded, honeycomb-structured carbon allotropes. The intensity ratios of the D to G peak ( I D / I G ) measure the degree of disorder in the carbon network. The I D / I G for our directly grown GraNRs is ~0.76, which is lower than the I D / I G of~1–6 reported for GraNRs etched from exfoliated graphene [37] . In transferred CVD graphene, the D peak is not present, owing to low defect density. For laterally confined graphene structures, the D band is commonly observed because of the increased contribution of graphene edges [37] . The I D / I G increases as the width of the GraNRs decreases, because of higher contribution of the edge effect [37] . Our directly grown GraNRs exhibit broadened D and G peaks, with full-width half-maximum of 100 and 62 cm −1 , respectively, implying disorder in the carbon network. A strong signature for single-layer graphene is the two-dimensional peak at 2,680 cm −1 . However, for GraNRs with widths <10 nm, this feature is suppressed (see Supplementary Fig. S8 ) [37] , [38] . 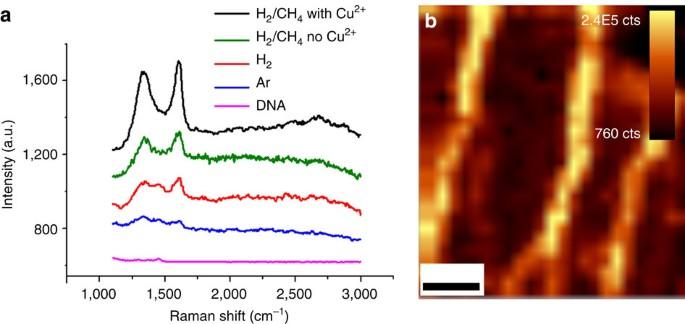Figure 3: Raman characterization showing conversion of DNAs into GraNRs. (a) Stretched lambda DNA (pink), 1,000 °C with Ar (blue), 1,000 °C with H2(red), SGP without Cu2+(green) and the SGP (black). (b) Raman mapping of the G band from SGP. Scale bar, 1 μm. Figure 3: Raman characterization showing conversion of DNAs into GraNRs. ( a ) Stretched lambda DNA (pink), 1,000 °C with Ar (blue), 1,000 °C with H 2 (red), SGP without Cu 2+ (green) and the SGP (black). ( b ) Raman mapping of the G band from SGP. Scale bar, 1 μm. Full size image A Raman spectrum was obtained for DNAs without Cu 2+ ions treated with Ar ( Fig. 3a , blue) or H 2 at 1,000 °C ( Fig. 3a , red). Although AFM showed that nanofibres were present in both cases (see Supplementary Fig. S9 ), the Raman spectra did not exhibit either D or G peaks, suggesting that the fibres were likely amorphous carbon. For H 2 -only ( Fig. 3a , red) and SGP without Cu 2+ conditions ( Fig. 3a , green), the intensity of the D and G peaks was weak, indicating a significant decrease in graphitic content. The Raman is in correspondence with the XPS showing that a significant amount of sp 2 carbon is formed only for metalized DNA exposed to SGP. It is likely that some sp 3 carbons or amorphous sp 2 carbons remain in the structure, and the term GraNR is appropriate. To confirm that the Raman signal could indeed be assigned to the GraNRs and not random sp 2 carbon contaminants, a two-dimensional G-peak Raman map was taken over a 5 × 5-μm scan area ( Fig. 3b ). Although the GraNRs were on a rough background with a lot of organic deposit, the deposits did not contribute to the Raman signal (see Supplementary Fig. S10 ). Interestingly, it was observed that the background became cleaner in the post-Raman characterization. This can be attributed to the laser burning away the organic deposits, whereas leaving the GraNRs intact. The zoom in phase image (see Supplementary Fig. S10d ) shows that the GraNRs are clearly intact after exposure to the laser. However, because of image roughness, an accurate analysis of the thickness changes could not be carried out. TEM characterization of GraNR structures To understand the extent of GraNR crystallinity, as well as definitively confirm the presence of graphene domains, we carried out high-resolution transmission electron microscopy (TEM) experiments. Owing to difficulties in transferring the as-grown GraNRs to a TEM grid, the direct growth of GraNRs suspended over a holey membrane was carried out. The process is challenging, as the growth process can result in a loss of GraNR integrity, leading to a collapse of the ribbon. We overcame this challenge by suspending thicker DNA over a holey Si 3 N 4 TEM grid. In this configuration, we could occasionally observe suspended nanoribbons across the hole. The typical width of observed nanoribbons was between 10 and 50 nm ( Fig. 4a ). The increased thickness was expected owing to the choice of thicker DNA bundles. At the edge of the nanoribbons, we clearly saw the lattice fringes with 0.34 nm spacing ( Fig. 4b ), consistent with interlayer distance in graphitic structures. This strongly indicates that we have successfully synthesized GraNRs containing regions of graphitic and amorphous carbon. 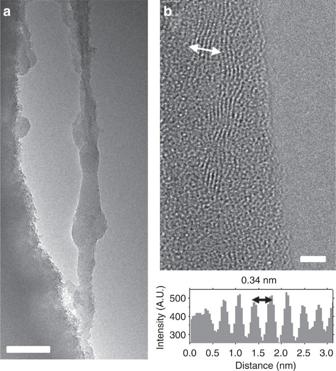Figure 4: TEM of GraNRs suspended over a holey Si3N4membrane. (a) GraNR suspended over a hole in the membrane. Scale bar, 50 nm (b) High resolution image of the GraNR showing the 0.34-nm lattice spacing consistent with interlayer stacking of graphene within the GraNR. Scale bar, 2 nm. Figure 4: TEM of GraNRs suspended over a holey Si 3 N 4 membrane. ( a ) GraNR suspended over a hole in the membrane. Scale bar, 50 nm ( b ) High resolution image of the GraNR showing the 0.34-nm lattice spacing consistent with interlayer stacking of graphene within the GraNR. Scale bar, 2 nm. Full size image Electrical characterization of GraNR structures To prepare GraNR-based electrical devices, we used 100 nm Si 3 N 4 on silicon, which provided an expanded thermal window for GraNR growth without dielectric degradation [39] . The electrical performance of the GraNRs synthesized utilizing SGP was measured by fabricating three-terminal back-gated FETs ( Fig. 5a and see Supplementary Fig. S11 ). The yield of the devices was high (~90%). Failure was typically because of pinholes in the dielectric, preventing device characterization. However, all characterized devices demonstrated sustained current, implying that continuity of the GraNRs was achieved on the ~5 μm scale. In contrast, the nanofibres obtained from annealed DNAs without Cu 2+ ions were non-conducting, confirming that the DNAs are converted to GraNRs only in the presence of metal ions. However, utilizing Si 3 N 4 as the dielectric only gave rise to metallic GraNRs. The I DS − V DS curve of the GraNR device is shown in Fig. 5b , with conductivity estimated to be 6.7 S cm −1 . This value is several orders of magnitude lower than the conductivity of lithographically etched GraNRs, suggesting that our GraNRs contain defects (for example, sp 3 carbons) or amorphous sp 2 carbon regions. We additionally evaluated the device in a three-terminal FET architecture (see Supplementary Fig. S12 ). The transfer plot showed p-type transistor behaviour with the Dirac point at +7 V (ref. 6 ). The conducting property of the GraNRs was further confirmed by molecular n -type charge-transfer doping to give n-type GraNR transistors with a Dirac point shifted to −10 V. The on/off ratio in the p -type GraNR device was approximately three, whereas the n-type device was approximately two. The detailed characterization of doping is provided in the Supplementary Note 1 . 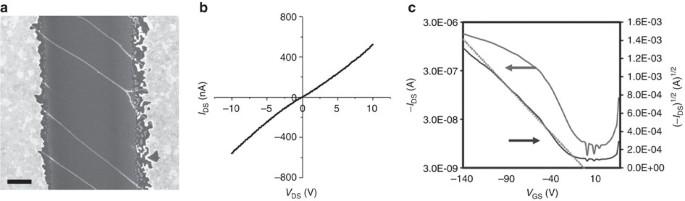Figure 5: Electrical analysis of GraNRs. (a) SEM of GraNRs bridging electrodes. Scale bar, 1 μm. (b)IDS−VDSplot for the metallic GraNRs. (c) Transfer plot of the semiconducting GraNRs functioning as a FET measured at 73% relative humidity and 35 °C. Figure 5: Electrical analysis of GraNRs. ( a ) SEM of GraNRs bridging electrodes. Scale bar, 1 μm. ( b ) I DS − V DS plot for the metallic GraNRs. ( c ) Transfer plot of the semiconducting GraNRs functioning as a FET measured at 73% relative humidity and 35 °C. Full size image During our studies on the influence of the growth conditions on the behaviour of the GraNRs in electrical devices, we fabricated FETs utilizing SiO 2 as the gate dielectric. The use of SiO 2 necessitated that the growth temperature be kept to a maximum of 800 °C to avoid increased leakage associated with the thermal breakdown of the dielectric. The resulting electrical behaviour of the GraNRs was found to significantly depend on the temperature and humidity of the environment. At standard laboratory conditions, the GraNRs were mostly insulating. However, when the devices were subsequently characterized under elevated humidity and temperature, we found that the conductivity of the GraNRs significantly increased. At 73% relative humidity and 35 o C, the devices demonstrated peak I DS of 1–10 μA. Moreover, the devices behaved as semiconductors with on/off ratios between 100 and 500 (see Supplementary Figs S13 and S14 ). We hypothesize that this effect is due to both an increase in the conductivity of the sp 3 portion as well as an increase in the bandgap of the graphitic sp 2 portion of the GraNRs [40] , [41] , [42] , [43] . An exemplary device using the semiconducting GraNRs showing a mobility of 0.21 cm 2 V −1 s −1 and an on/off ratio of 192 is shown in Fig. 5c . Owing to the significantly improved on/off ratios, the devices were termed semiconducting. The detailed characterization of the semiconducting devices is provided in the Supplementary Note 2 . In this paper, we have demonstrated a bottom-up synthesis method of aligned GraNRs using a DNA template. The arrangement of the DNA is tuneable allowing access to cross-bar architectures from two perpendicularly aligned DNA bundles [28] , [44] ( Fig. 1d ) or potentially exotic structures via DNA origami [30] . The facile transfer of DNA patterns (that is, cross-bar DNA stamps) means that DNAs can be placed into ordered arrays or within pre-determined patterns (for example, circuit layout) over large areas [45] , thereby opening the way for large-scale production of graphene-based nanoribbon FETs. The ability to align the DNAs on the surface before growth negates the need for post-growth assembly. Moreover, DNA provides a convenient platform for the exchange of metal catalysts or base-pair structures, leading to desired shapes and functionalities of the carbon architectures [46] . Characterization of the as-grown GraNRs suggests that the nanoribbons consist of a mixture of graphitic and amorphous carbon domains. These results are supported by the high-resolution TEM images, as fringes clearly corresponding to interlayer distance in graphitic structures are observed. The combination of graphitic and amorphous carbon is supported by XPS results as well as conductivity measurements within FETs. Interestingly, the use of SiO 2 as the dielectric resulted in the formation of semiconducting GraNRs. We attribute the semiconducting behaviour of the resulting ribbons to a surface effect on the catalytic growth mechanism of GraNRs. We hypothesize that the use of a SiO 2 surface results in higher-quality graphitic regions, intermixed with regions of amorphous carbon, akin to islands of nanoscale graphene within an amorphous carbon ribbon. The amorphous carbon ribbons behave as resistors in series with the graphitic regions of the GraNRs. Thus, a gating of the graphitic regions is observed, in series with large channel resistance provided by the amorphous carbon. The additional channel resistance imparted by the regions of amorphous carbon may explain the high voltages used to drive the GraNRs. In GraNRs grown on Si 3 N 4 , the ribbon contains increased graphitic character; however, it is of lower semiconducting quality. In these ribbons, conducting behaviour is observed, utilizing lower voltages. Although the exact mechanism of GraNR growth is unknown, we believe that this provides critical evidence on the impact of surface chemistry on nanoscale ribbons growth. Mechanistic understanding of GraNR growth, quantification of the defect/amorphous carbon content and improvements in the crystalline graphene content are expected to significantly increase GraNR device performance. In the future, although further improvements in growth and understanding of the mechanism are needed, our method opens up a new direction for the direct growth of GraNRs. The catalysed growth of graphene via reduction of metal salts will undoubtedly result in novel carbon architectures. Future work on the characterization of GraNRs with atomic resolution scanning tunnelling microscopy will provide insight into edge structures and growth mechanisms. Finally, the use of growth conditions similar to CVD graphene may be used to prepare both electrodes and semiconductors in a single step, leading to direct growth of all-graphene integrated circuits. Materials Phenyltrimethoxysilane (PTS), aminopropyltriethoxysilane (APTES) (Gelest), trimethylamine, 99% (Fisher Scientific), SiO 2 and Si 3 N 4 wafers, Lambda DNA (New England Biolabs), copper nitrate (ACROS), PELCO 8 nm silicon dioxide membrane TEM grid (Ted Pella), 2-( N -morpholino)ethanesulfonic sodium salt (Sigma), Sylgard Silicone Elastomer Kit (Dow Corning) were used as received. PTS modification of SiO 2 and Si 3 N 4 wafers The 300 nm silicon dioxide and 100 nm silicon nitride wafers were exposed to oxygen plasma at 150 W, 250 mTorr, for 5 min. The wafers were then immersed in a 0.3% (v/v) PTS and 15% (v/v) triethylamine solution in toluene for 16 h. The wafers were rinsed and sonicated in toluene two times to remove the non-covalently attached molecules. Preparation of DNA templates MES buffer (50 mM) is prepared by dissolving 2-( N -morpholino)ethanesulfonic sodium salt in deionized water and adjusting the pH to 5.5 using sodium hydroxide. Lambda DNA was diluted in MES buffer to 30 μg ml −1 with 30 mM NaCl. The DNA solution is dispensed onto the chips and incubated for 2 min before spin coating at 1 krpm for 30 s. The substrates are then immersed in 0.1 M Cu(NO 3 ) 2 for 5 min. As the substrate is quite hydrophobic, the solution de-wets from the substrate and no rinsing is required. DNA film The 300-nm silicon dioxide chips were exposed to oxygen plasma. A 500 μg ml −1 DNA solution was dispensed onto the chip and spin-coated at 3 krpm. The wafer was briefly rinsed with deionized water to remove the residual buffer salts. The AFM image of the film is shown in Supplementary Fig. S1 . CVD process The wafers were placed into a single-zone furnace and exposed to CVD growth conditions. First, the furnace was raised to 1,000 °C under a hydrogen flow of 8 sccm at 90 mTorr, it was further kept at 50 mTorr for 30 min to reduce the copper ions intercalated in the DNA. In the growth step, methane and hydrogen were flowed at 8 and 10 sccm, respectively, at a pressure of 50 mTorr. The temperature was kept at 1,000 °C for 30 min. Lastly, the furnace was cooled down to room temperature; the hydrogen flow was kept at 8 sccm at 50 mTorr. This process is hereinafter denoted as our SGP. Other growth processes were performed to understand the growth mechanism of the GraNRs. To study the need of methane gas, the standard growth was performed but with the growth step eliminated (denoted as H 2 only). To study the need for hydrogen in reducing the copper, an experiment in an overpressure argon environment was carried out (denoted as Ar only). The duration and pressure in each step were kept similar to the SGP unless stated. The details of the processes are tabulated in Table 1 . Fabrication of GraNR devices The electrical performance of the GraNRs was measured by fabricating three-terminal back-gated FETs with gold as the source/drain contacts, deposited by thermal evaporation through a conforming parylene shadow mask [47] ( Fig. 4a ; Supplementary Fig. S9 ). The channel lengths were 5 μm and the widths were 100 μm. The orientations of the GraNRs were confirmed with AFM before electrode alignment. Electrical characterization of the devices was carried out using a semiconductor analyser (Keithley 4200-SCS). For the devices on Si 3 N 4 , termed metallic GraNRs, the typical density of GraNRs observed with AFM was estimated to be 60 GraNRs bridging a single electrode. We assumed that each GraNR has a width of 10 nm and height of 0.7 nm, aligned perpendicularly to the electrodes. From this, the GraNR conductivity is estimated to be about 6.7 S cm −1 . For the FET devices, the width of the device was estimated to consist of 60 GraNRs with a width of 10 nm each, or W =600 nm. As the L of the electrodes used was 5 μm, the W / L was estimated to be 0.12. For the devices on SiO 2 , termed semiconducting GraNRs, the typical density of GraNRs observed with AFM was estimated to be 50 GraNRs bridging a single electrode. We assumed that each GraNR has a width of 10 nm, or W =500 nm. As the L of the electrodes used was 5 μm, the W / L was estimated to be 0.1. Doping of GraNR Functionalization was done by spin coating 5 mg ml −1 2-(2-methoxyphenyl)-1,3-dimethyl-1H-benzoimidazol-3-ium (O-MeO-DMBI) ethanolic solution onto the surface of as-prepared GraNR devices. This was followed by annealing at 100 o C for 1 h to remove the physisorbed oxygen and water molecules. All the processing and measurements were performed in a nitrogen-filled glove box. Transmission electron microscopy We utilized aberration-corrected TEM to study the width of the GraNRs. Unfortunately, we were not able to transfer the GraNRs from the growth substrate, presumably owing to the small surface area of the ribbon and the strong interaction with the substrate. Thus, the GraNRs were grown directly on an 8-nm thick SiO 2 membrane TEM grid. The width of the GraNR measured about 10 nm ( Supplementary Fig. S1A ). PELCO 8 nm silicon dioxide membrane TEM grid (Ted Pella) was used for the TEM imaging experiments. The TEM grid was modified with APTES by immersing it in a 0.5% (v/v) solution in anhydrous toluene for 1 h in the glove box. The grid was then rinsed gently by dipping into toluene and wicked dry. The metalized DNA was transferred onto the grid from PDMS instead of spin coating so as to minimize damage to the membrane. DNA was spin-coated onto PDMS and metalized with 0.1 M copper nitrate for 5 min. The DNA was transferred onto the support film by using a drop of ethanol to ensure good contact between the membrane and PDMS. The grid was then exposed to the SGP. For imaging the suspended GraNRs, a holey Si 3 N 4 TEM grid (PELCO, 200 nm membrane with 2.5 μm holes) was O 2 plasma treated for 5 min and then soaked into a diluted APTES solution (100 μl APTES dissolved in 3 ml anhydrous toluene for 1 h in the glove box). The grid was then rinsed gently by dipping into toluene and wicked dry. A droplet of lambda DNA was coated onto the modified TEM grid and gently blown away along a single direction. Before CVD growth, this TEM grid was soaked in 0.1 M Cu(NO 3 ) 2 solution for a period of 5 min. The grid was the exposed to the SGP. TEM imaging was performed at 80 kV using a FEI Titan equipped with a spherical aberration (Cs) corrector in the image-forming (objective) lens. The Cs coefficient was set to approximately −10 μm. The images were acquired using an Ultrascan 1,000 CCD camera. For additional TEM studies, a Zeiss Libra 120 with an in-column energy filter was used at 120 kV. Scanning electron microscopy SEM was performed with an FEI Magellan 400 XHR scanning electron microscope operated at 20 kV. Additional SEM images in Supplementary Fig. S3 . Atomic force microscopy AFM was performed using a Digital Instruments Nanoscope IV operated in tapping mode. Super sharp silicon tip and standard point probes (Nanosensors), with typical tip radius curvature of 2 and 7 nm, respectively, were used. Additional AFM images in Supplementary Fig. S1 . Raman characterization Raman was carried out with a WITec system with a 532-nm source and a laser power of 4 mW. An × 100 objective lens with a numerical aperture=0.95 was used with an estimated spot size of 683 nm. The mapping was set to scan size of about 5 × 5 μm and the pixel size is 250 nm. The stage movement and data acquisition were controlled using ScanCtrl Spectroscopy Plus software from WITec GmbH, Germany. The integration time for each scan is 10 s, and the peak intensity was normalized. Data analysis was done using WITec Project software. X-ray photoelectron spectroscopy XPS was carried out with PHI 5000 Versaprobe equipped with monochromatic Al Kα source, pass energy of 1,486.6 eV and a step size of 0.1 eV. The samples were prepared on SiO 2 , and all the spectra were referenced to the Si 2 p peak in SiO 2 with binding energy of 103.3 eV. How to cite this article: Sokolov, A. N. et al. Direct growth of aligned graphitic nanoribbons from a DNA template by chemical vapour deposition. Nat. Commun. 4:2402 doi: 10.1038/ncomms3402 (2013).